On “Coherent control in the extreme ultraviolet and attosecond regime by synchrotron radiation” by Hikosaka et al,Nat. Comm. 10, 4988 (2019) 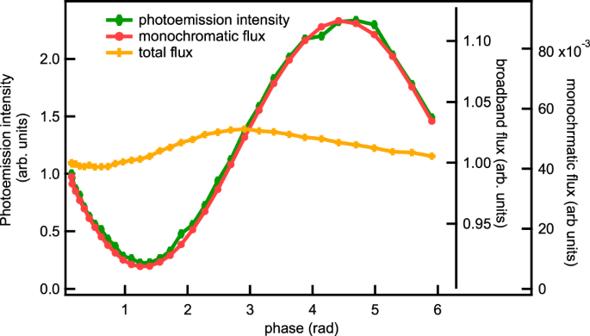Fig. 1: Measured resonant photoemission intensity at binding energy 2.5 eV (green curve), monochromatic flux (red curve) and total flux (orange curve) as a function of phase. The photoemission intensity and monochromatic flux are plotted on different axes from zero and scaled so the maxima overlap. Both curves vary from 10% to 100% of the maximum. Note the expanded scale for the total flux: the flux varies from 97% to 100% of the maximum. Photon energy: 38 eV. 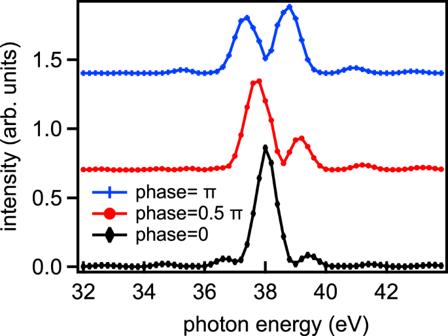Fig. 2: Measured spectral intensity as a function of photon energy with the undulator gaps optimised for 38 eV emission, and three values of the phase setting. Lower curve: phase = 0 rad; centre curve, phase = 0.5π rad; top curve, phase = π rad. The experiments were carried out at the Nanospectroscopy beamline [10] , [11] at the Elettra synchrotron light source. The photon source consists of two identical Sasaki Apple II type undulator sections (each with 20 periods and period length 10 cm) and a phase shifter electromagnet between them [12] , [13] , [14] . This arrangement is similar to that of Hikosaka et al. [1] , [2] , who used a pair of undulators with 10 periods each. The energy of the electrons in the storage ring was 2.4 GeV, and the average electron bunch duration was ~60 ps. The light beam was spatially defined by an aperture of 0.5 mm (horizontal) by 0.9 mm (vertical) at a distance of 10 m from the source point in the second undulator. The experimental station consists of a photoemission microscope [10] . The sample was the (0001) surface of a single crystal of Rhenium. The Re crystal was cleaned by repeated annealing cycles to about 1100 °C in molecular oxygen (P O2 = 1 × 10 −6 mbar), followed by a high temperature flash (to about 2000 °C) under ultrahigh vacuum conditions. We measured the resonant photoemission of the valence band of Re. The resolving power (E/ΔE) of the monochromator was ~10 4 for the photon energies considered. The photoelectron energy analyser of the photoemission microscope has an energy resolution of about 150 meV under typical operation conditions [10] . In the range from 35 to 45 eV photon energy, the 5d electrons of the valence band display resonant enhancement with a Fano line profile. The two paths leading to the interference are direct ionisation, and resonant excitation of the 4f 5/2,3/2 electrons to the unoccupied states, followed by autoionization; both paths yield the same final state. The total flux from the beamline as a function of phase was measured by setting the monochromator to zero order and inserting a photodiode into the beam after the exit slit, but before the experimental station. The monochromatic flux as a function of phase was also measured with the same photodiode. Identical phase scans were performed to measure the diode signal, and then to measure the resonant photoemission signal from the sample with the diode removed. The theoretical data in Supplementary Fig. 2 were calculated using the program Spectra [13] , [15] .